Laser-targeted photofabrication of gold nanoparticles inside cells Nanoparticle manipulation is of increasing interest, since they can report single molecule-level measurements of the cellular environment. Until now, however, intracellular nanoparticle locations have been essentially uncontrollable. Here we show that by infusing a gold ion solution, focused laser light-induced photoreduction allows in situ fabrication of gold nanoparticles at precise locations. The resulting particles are pure gold nanocrystals, distributed throughout the laser focus at sizes ranging from 2 to 20 nm, and remain in place even after removing the gold solution. We demonstrate the spatial control by scanning a laser beam to write characters in gold inside a cell. Plasmonically enhanced molecular signals could be detected from nanoparticles, allowing their use as nano-chemical probes at targeted locations inside the cell, with intracellular molecular feedback. Such light-based control of the intracellular particle generation reaction also offers avenues for in situ plasmonic device creation in organic targets, and may eventually link optical and electron microscopy. Gold nanoparticles are proving to be a powerful tool to probe cell function and behaviour [1] , [2] . The unique properties of gold allow tagging of cellular components, local amplification of the excitation light field or dynamically reporting the positions and chemical compositions of compounds near the probe [3] , [4] . While surface-enhanced Raman spectroscopy has enormous potential for quantifying biochemical phenomena within living cells, a major limitation has been the placement of nanoparticles at locations of interest. Without controlling the locations of particles, useful information is still gained, where particles uptaken by normal pathways in the cell can function as a type of nano-endoscope [3] , but there is significant interest in methods to control the uptake pathways and final destinations of nanoparticles in cells. Typical methods involve using conjugate tags with the particles, injecting the particles by micropipette, attaching particles to a nanopipette [5] or optimizing particle coatings to modulate typical cell–particle interaction pathways [6] , [7] . However, there are several limitations with these methods; bare nanoparticles do not readily penetrate cellular membranes, and even once inside the cell, they cannot move freely. A promising alternative has been to grow gold nanoparticles within bacteria [8] , [9] , [10] , [11] or human cells by infusion of a low-density chloroaurate solution [12] , [13] , albeit without the means to control location. Here we demonstrate a new approach that allows both subcellular penetration and precise control of nanoparticle placement. The cells are infused with a solution of gold salts, which penetrate cellular membranes. Then, using a focused laser beam controlled by scanning mirrors, we directly fabricate nanoparticles by photoreducing the solution to gold particles, with the reduction occurring in a near diffraction-limited spot. The gold ion solution can then be washed out, while fabricated nanoparticles remain within the cell. Surprisingly, the nanoparticles are formed as pure gold crystalline structures, and fabricated nanoparticles remain at the original irradiation site without significant diffusion. The size of fabricated nanoparticles ranged from 2 to 20 nm, and can be formed anywhere within the cell. Such small particles do not usually lead to the observation of surface-enhanced Raman scattering (SERS), but aggregated particles are observed in the laser focal area, and SERS can be successfully generated from these fabricated regions. The spatial control of the reaction is clear enough that text can be enscribed in gold inside the cells. This study demonstrates a new direction for creating gold nanoparticles or nanostructures of interest at locations of interest inside a cell without the use of coatings or conjugate chemistry, and could underpin new applications in the control of nanoparticles and plasmonics within cells. 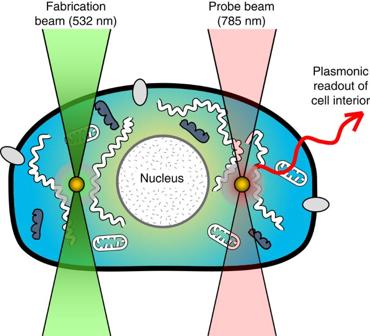Figure 1: Photoreduction of aqueous gold solution by targeted laser beam. While nanoparticles do not freely pass through a cell, the cell is permeable to gold ion solution. By infusing the cell culture dish with gold ion solution, focused 532-nm irradiation can then trigger photoreduction at an area of interest and ionic gold can later be washed out, leaving permanent fabricated gold nanoparticles at the laser focus. Intracellular spectra can then be studied by Raman spectroscopy, without luminescent interference, using near-infrared light excitation (785 nm). Proof of particle fabrication Figure 1 shows a schematic overview of the process (see Methods section for details). In overview, the combination of millimolar concentrations of HAuCl 4 gold solution and several milliwatts of 532 nm irradiation, focused at an intracellular location of interest is sufficient to produce pure gold crystal nanoparticles by photoreduction. Following irradiation of the cell, brightfield images of the area where the laser was focused revealed black regions ( Fig. 2a ), while areas not irradiated retained their original contrast, and control experiments without HAuCl 4 did not produce dark regions. This contrast change was quantified by measuring the change in brightfield intensity before and after irradiation at different laser powers and exposure times ( Fig. 2b ), with control experiments shown in Fig. 2c . While it might be expected that the photoreduction of gold would depend on the location in the cell, experiments carried out in cells at randomly chosen locations ( n =30 for each parameter) all show some darkening of the target area, regardless of the subcellular location. In all experiments, laser power of 1.3 mW (corresponding to 11.2 mW μm −2 , assuming diffraction-free focusing and 1/e 2 criteria for spot size) and 3 s exposure time consistently produced a gold-ion-dependent contrast change in the cell. While brightfield imaging alone does not prove the existence of gold nanoparticles, it provides several concrete conclusions. First, the observed change in brightfield intensity is reproducible. Second, it occurs only inside the cell, and third, requires the presence of gold ion solution. In contrast, control experiments ( Fig. 2c ) lacking gold ion solution, laser irradiation, a cell target or any combination thereof, resulted in no contrast change. In separate experiments, 785 nm irradiation of the same samples with up to 180 mW for 120 s did not produce evidence of particles. It is clear then, that the dark regions are due to the combination of 532 nm light, gold ions and the cellular environment. With a continuous wave 532-nm laser wavelength, the photon absorption mode should not be significantly nonlinear [14] , and the brightfield image contrast changes shown in Fig. 2 are approximately linear for 0.8 and 1.3 mW, and show some evidence of saturation for 1.7 mW. If significant nonlinearity was present, we should expect to see stronger contrast change, with the height of the bars in Fig. 2 curving upwards with increasing power and/or exposure time. We next employed electron microscopy to analyse the content of the fabricated regions. Figure 1: Photoreduction of aqueous gold solution by targeted laser beam. While nanoparticles do not freely pass through a cell, the cell is permeable to gold ion solution. By infusing the cell culture dish with gold ion solution, focused 532-nm irradiation can then trigger photoreduction at an area of interest and ionic gold can later be washed out, leaving permanent fabricated gold nanoparticles at the laser focus. Intracellular spectra can then be studied by Raman spectroscopy, without luminescent interference, using near-infrared light excitation (785 nm). 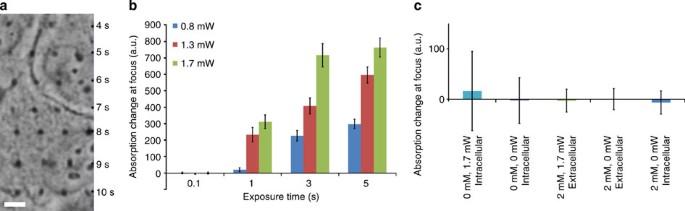Figure 2: Fabrication of nanoparticles inside the cell. (a) Brightfield image array of black spots resulting from laser irradiation of cells incubated with 2 mM HAuCl4with 0.3 mW for increasing exposure times of 4 s (top row) to 10 s (bottom row). Scale bar, 4 μm. Absorption change due to irradiation of gold ion-infused cells is quantified inb, and control experiments (c) show that the laser-induced change occurs only inside the cell (intracellular), only in the presence of gold ion solution, and only with laser light. If the cells were producing a comparable amount of nanoparticles by endogenous processes, the 0-mW columns incwould be comparable to those inb. The change is shown in a.u., but experimentsbandcare directly comparable in numerical value. Error bars are the s.d. andn=30 for each parameter. Full size image Figure 2: Fabrication of nanoparticles inside the cell. ( a ) Brightfield image array of black spots resulting from laser irradiation of cells incubated with 2 mM HAuCl 4 with 0.3 mW for increasing exposure times of 4 s (top row) to 10 s (bottom row). Scale bar, 4 μm. Absorption change due to irradiation of gold ion-infused cells is quantified in b , and control experiments ( c ) show that the laser-induced change occurs only inside the cell (intracellular), only in the presence of gold ion solution, and only with laser light. If the cells were producing a comparable amount of nanoparticles by endogenous processes, the 0-mW columns in c would be comparable to those in b . The change is shown in a.u., but experiments b and c are directly comparable in numerical value. Error bars are the s.d. and n =30 for each parameter. Full size image Transmission electron microscopy of fabricated nanoparticles Owing to the difficulty in locating a three-dimensional resolved target spot inside one cell, cells for electron microscopy were irradiated by a line focus pattern passing through the cell so that the laser focus was parallel to the sample dish. The laser power in line mode is comparable to the single-point mode used above. The transmission electron microscope (TEM) images in Fig. 3 show the formed particles. 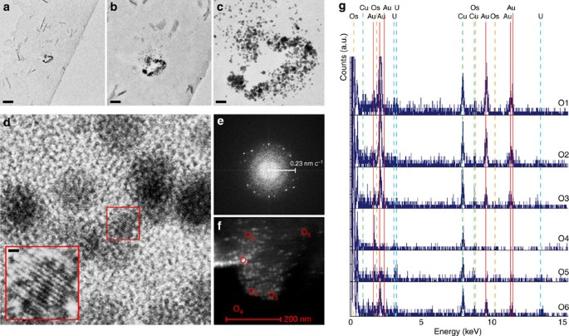Figure 3: Electron microscopy images and X-ray dispersive analysis of fabricated particles. (a–c) Laser focus region with aggregation of nanoparticles. (d) High-resolution image of single particles. The gold crystal lattice is visible (see enlarged inset). The lattice spacings are measured by spatial frequencies in the Fourier transform shown ford, shown ine, and corresponds to the 2.35-Å interplanar spacing of gold. (f) Scanning transmission darkfield electron microscopy, with X-ray dispersive analysis ingconfirming the signature of gold with Au peaks marked in red. Other heavy metals appear from the sample preparation (osmium, uranium) and copper appears from the substrate. Together, these results show that the particles fabricated by laser range in size from 2 to 20 nm and are composed of pure gold crystals, based on the X-ray analysis and lack of inclusions observed in the lattices. The distribution of nanoparticles inbappears to be confined to a region of ~340 nm in diameter. Scale bars for (a–c) are 310, 136 and 39 nm, respectively, while the inset scale bar fordis 0.54 nm. Figure 3a shows the cell outline, with a dark region representing the laser focus with progressively larger zoomed images ( Fig. 3b,c ). The periodicity of the lattice structure inside the nanoparticles in the highest-resolution (HR)-TEM image ( Fig. 3d ) is ~0.23 nm, and Fourier analysis shows a number of points at a periodicity of 0.23 nm per cycle or slightly higher ( Fig. 3e ), with an average of 0.227 nm. As a face-centred cubic crystal with a lattice constant of 0.408 nm (ref. 15 ), the highest density d 111 plane for pure gold will have an interplanar spacing of 0.235 nm, and a slightly tighter spacing is to be expected to be measured in the TEM images since the crystal orientation should not be perfectly aligned with the imaging plane. X-ray diffraction analysis of 1 mM HAuCl 4 solution in a bath application on HEK293 cells over long periods of time in a previous report [13] has also primarily shown the d 111 peak as evidence of gold. No inclusions or crystal defects are apparent in the formed particles, leading to the conclusion that the crystals are formed from only one atomic source, that is, only one metal, and that the fabrication process is not contaminated by molecules from the cellular environment. Further confirmation that the metal in the lattice structures is gold was demonstrated using the high-angle annular dark-field-scanning TEMmode ( Fig. 3f ), which shows particles on a dark background. Selected regions are then measured by energy-dispersive X-ray analysis, where heavy metals appear as peaks in the energy spectrum on the x axis ( Fig. 3g ). Peak assignments are from the TEM microscope library. The results show a number of peaks that confirm the presence of gold. Uranium, osmium and copper are also used in the TEM sample preparation process and appear along with the characteristic gold bands. Figure 3: Electron microscopy images and X-ray dispersive analysis of fabricated particles. ( a – c ) Laser focus region with aggregation of nanoparticles. ( d ) High-resolution image of single particles. The gold crystal lattice is visible (see enlarged inset). The lattice spacings are measured by spatial frequencies in the Fourier transform shown for d , shown in e , and corresponds to the 2.35-Å interplanar spacing of gold. ( f ) Scanning transmission darkfield electron microscopy, with X-ray dispersive analysis in g confirming the signature of gold with Au peaks marked in red. Other heavy metals appear from the sample preparation (osmium, uranium) and copper appears from the substrate. Together, these results show that the particles fabricated by laser range in size from 2 to 20 nm and are composed of pure gold crystals, based on the X-ray analysis and lack of inclusions observed in the lattices. The distribution of nanoparticles in b appears to be confined to a region of ~340 nm in diameter. Scale bars for ( a – c ) are 310, 136 and 39 nm, respectively, while the inset scale bar for d is 0.54 nm. Full size image Fabricated nanoparticle position stability and aggregation While fixation was necessary for the TEM observation, experiments using brightfield (absorption) imaging showed no dispersion of dark regions over time periods of up to 30 min. Nanoparticles are often observed to relocate inside a cell over such a time frame [16] , however, these results indicate that even when nanoparticles are formed in situ , without containment by endocytotic vesicles, their position remains stable. While this could be explained by the nanoparticles being seeded on cellular structures and remaining attached to them, the HR-TEM images show that the nanoparticles are, at least initially, composed entirely of gold atoms without inclusions or defects. This suggests that their positional stability may result from restriction of the movement by cellular structures. Although larger nanoparticle sizes are usually used with endocytosis-based particle entrance methods, the nanoparticles produced by the photoreduction methods are potentially more stable, since they can be fabricated in regions that particles cannot penetrate or escape from. This represents a unique benefit in addition to the property of not requiring surface coatings or treatment to reach a target location. To properly demonstrate that control of the nanoparticle fabrication region could be achieved, the laser focus was also scanned through the cell in a predetermined pattern, showing that arbitrary photoreduction regions could be generated. 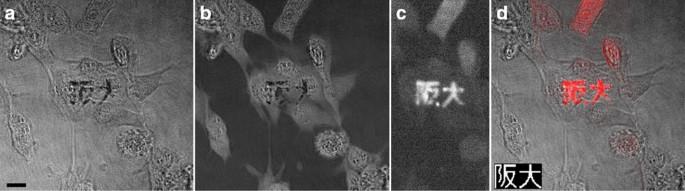Figure 4: Phase and spectroscopic imaging of photofabricated characters in gold inside cells. Absorption imaging (a) and phase imaging (b) by digital holographic microscopy (DHM) show the fabricated pattern to some degree, but the luminescence image taken via an imaging spectrometer (c) shows the pattern most clearly. An overlay (d) shows luminescence in the red channel on top of the absorption image (greyscale), with the small inset showing the actual scan pattern for the gold fabrication. The results show that locations of interest can be targeted for photofabrication. Scale bar, 12 μm. Figure 4 shows the result of a laser focal scan pattern using the characters for the name of our host institution (Osaka University). In addition to the laser focal scan pattern, we constructed a simultaneous multimodal optical system for monitoring sample absorption and phase by digital holographic microscopy (DHM), and luminescence or other spectral signals [17] . The results show that the nanoparticle photoreduction regions are readily visible in the absorption image, but only barely visible in the phase-imaging mode. This is expected since the phase change due to small particles of a complex refractive index should be relatively low. The luminescence signal is clearer than either the absorption or phase modes, again consistent with the appearance of nanoparticles that can exhibit luminescence from sub-wavelength particles. The luminescence channel also includes autofluorescence from the cell, which occupies a similar spectral range to the particle luminescence, and some cells appear stronger than others in this channel. However, cells exhibiting a stronger signal in the luminescence channel near the edge of the sample, away from the targeted pattern, do not show any corresponding change in absorption or phase, indicating they are not luminescence signals from nanoparticles. Figure 4: Phase and spectroscopic imaging of photofabricated characters in gold inside cells. Absorption imaging ( a ) and phase imaging ( b ) by digital holographic microscopy (DHM) show the fabricated pattern to some degree, but the luminescence image taken via an imaging spectrometer ( c ) shows the pattern most clearly. An overlay ( d ) shows luminescence in the red channel on top of the absorption image (greyscale), with the small inset showing the actual scan pattern for the gold fabrication. The results show that locations of interest can be targeted for photofabrication. Scale bar, 12 μm. Full size image While the ability to choose the location of interest for fabrication and target that area with the laser beam is the main motivation of the present study, it is also interesting to explore what happens when the entire sample is irradiated. 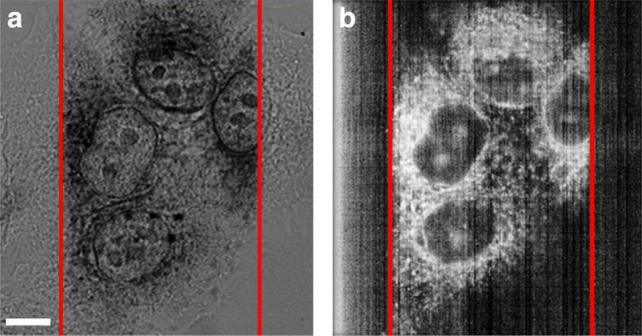Figure 5: Irradiation of the entire field of view produces nanoparticles throughout the cell. The cells are shown in brightfield (a) and luminescence (b). The particle generation in the irradiated region (between the red lines) is widespread but confined to the areas where laser light produced photoreduction. Note the cell on the right-hand side is bisected by the edge of the irradiation region but luminescence remains within the photoreduction region. When holding laser power and exposure constant, the effect appears stronger in the cytoplasm compared with the nucleus, while nucleolus regions appear stronger than the rest of the nucleus, indicating some spatial variability in photoreduction based on the microenvironment. The resulting spatial variation in nanoparticle generation has the potential to be used as a contrast agent in electron microscopy. Scale bar, 10 μm. Figure 5 shows the possibility of fabricating particles over large regions of the cell, which appear to remain in place after photoreduction. Several cells in the large central region of the entire field of view (marked by red lines) were irradiated by 532 nm irradiation. When irradiating entire cells, instead of single points, we use line-shaped irradiation and the total available intensity in such a setup is 0.6 mW μm −2 . The total exposure in Fig. 5 was then 1 s per line, repeated 10 times (for comparison, those in Fig. 2 were 1.7–6.9 mW μm −2 , for exposure times of 0.1 to 5 s). The results from irradiating the entire cells show that irradiating either a single point, or an entire line through the cell, with approximately comparable parameters, produces nanoparticle luminescence. Images were acquired by (a) brightfield and (b) luminescence microscopy, where the brightfield image shows absorption and the luminescence image shows gold-based luminescence from fabricated particles. Figure 5: Irradiation of the entire field of view produces nanoparticles throughout the cell. The cells are shown in brightfield ( a ) and luminescence ( b ). The particle generation in the irradiated region (between the red lines) is widespread but confined to the areas where laser light produced photoreduction. Note the cell on the right-hand side is bisected by the edge of the irradiation region but luminescence remains within the photoreduction region. When holding laser power and exposure constant, the effect appears stronger in the cytoplasm compared with the nucleus, while nucleolus regions appear stronger than the rest of the nucleus, indicating some spatial variability in photoreduction based on the microenvironment. The resulting spatial variation in nanoparticle generation has the potential to be used as a contrast agent in electron microscopy. Scale bar, 10 μm. Full size image Point-based illumination results show the potential to create particles at any location, and comparison with the line-irradiated production of nanoparticles indicates that the absorption and fabrication mechanism is approximately linear. However, the luminescence image in Fig. 5b shows that, for given laser irradiation conditions, the amount, shape or size of fabricated particles depend on the cellular location. By choosing appropriate irradiation conditions, these images also show the potential of using in situ fabrication for creating particles where the particle generation depends on the cellular environment and may consequently find use as a staining technique in electron microscopy. Nanoparticles appearing in the TEM images ( Fig. 3b ) appear to overlap each other, however, it should be noted that the TEM method produces a projection of all nanoparticles in the microtome section. Since the section thickness is 70 nm, much larger than the nanoparticle dimensions, the nanoparticles are not necessarily overlapped. Without inter-particle hotspots, and considering the small particle sizes, the particle distributions would be expected to produce weak or no SERS signals. We then used 785-nm wavelength irradiation to investigate the possibility of using the photofabricated particles to enhance Raman scattering from fabricated regions. SERS from fabricated particles A major application of nanoparticles in cell experiments is the measurement of SERS, because it provides detailed chemical information. However, due to the plasmon resonance effect [18] , it usually requires the use of much larger nanoparticles. To determine whether SERS could be observed in two-dimensional photofabricated imaging data requires searching through thousands or millions of spectra and determining whether each signal constituted a SERS signal or not. We therefore fabricated nanoparticle regions, imaged the resulting two-dimensional spectral distribution by 785-nm irradiation and recorded all data in a three-dimensional hyperspectral image. We then applied our recently developed method of automated detection and classification [19] to detect the presence of SERS spectra. 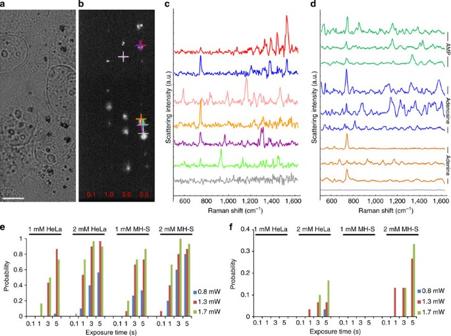Figure 6: Surface-enhanced Raman scattering from fabricated regions. While small nanoparticles do not usually provide a basis for surface-enhanced Raman measurements, point irradiation of 532 nm, 5 mW laser light for 0.1 to 5 produced regions shown in brightfield (a) and luminescence (b) where exposure times for each column of points are also denoted inbin red. The measurement of SERS signals was done by 785 nm light, where SERS data were automatically detected (see methods) to avoid bias. SERS was only detected from regions where 532 nm light was irradiated. SERS-generating locations are marked inbby +, with each corresponding spectra shown inc. SERS spectra of AMP, adenosine and adenine (three representative spectra for each) were also measured for comparison (d, see Methods for details). The horizontal axis shows Raman scattering shift in cm−1. Probabilities for the occurrence of luminescence and SERS from fabricated regions are shown ineandf, respectively, for varying laser power, exposure time, cell type and HAuCl4concentration (1 or 2 mM). Error bars are not shown; probabilities are number of occurences divided by number of trialsnwhere for HeLa cells,n=30 and for MH-S macrophages,n=15. Scale bar, 10 μm. Figure 6 shows the resulting regions in the cell (a), the corresponding luminescence (b) and the resulting spectra (c) for regions marked in Fig. 6b . Figure 6b also shows the exposure time in red for each set of points. The resulting spectra show a number of peaks in the fingerprint region, predominantly around 749 cm −1 , and between 1,300 and 1,500 cm −1 . Quantitative assignment of peaks is always challenging in SERS analysis of an inhomogeneous sample, but a number of peaks appear at locations consistent with biological molecules. Peaks at 830, 1,295, 1,316, 1,438 and 1,444 cm −1 are consistent with lipid components [20] , [21] , while 932, 968, 1,073, 1,159, 1,270 cm −1 are commonly seen in protein (amide) or amino-acid bands [22] , [23] . Nucleic acids such as adenosine and guanosine are also readily detected by SERS and although often observed closer to 730 cm −1 , the ring-breathing mode of adenosine is reported to undergo a shift, depending on the orientation to the SERS surface, and may be responsible for the strong peak around 749 cm −1 (refs 24 , 25 ). Cytochrome c and haeme-based compounds also show a strong peak near 750 cm −1 (ref. 26 ), however, other typical cytochrome c peaks were not observed. From these peak assignments, it appeared that adenine-based molecules may represent a significant part of the measured signal, and therefore the three most common forms of adenine found in a cell were separately measured using a preparation of commercially available 50-nm gold nanoparticles ( Fig. 6d , see Methods for details). The commercially available nanoparticles were used for these comparison reference measurements since the spectral measurement method presented in this report is itself new. Spectra were extracted by algorithm in the same manner as for fabricated nanoparticles. Adenine, with the addition of ribose to form adenosine, and the further addition of phosphate to form the nucleotide adenosine mono-phosphate all show a clear ring-breathing mode near 750 cm −1 , but these molecular spectra do not present the same peaks in the 800–1,600 cm −1 range in the fingerprint region observed from the fabricated regions. This indicates that, while the adenine-breathing mode appears to be present in fabricated regions, the photoinduced nanoparticles are reporting signals from molecules other than simply adenine. Figure 6: Surface-enhanced Raman scattering from fabricated regions. While small nanoparticles do not usually provide a basis for surface-enhanced Raman measurements, point irradiation of 532 nm, 5 mW laser light for 0.1 to 5 produced regions shown in brightfield ( a ) and luminescence ( b ) where exposure times for each column of points are also denoted in b in red. The measurement of SERS signals was done by 785 nm light, where SERS data were automatically detected (see methods) to avoid bias. SERS was only detected from regions where 532 nm light was irradiated. SERS-generating locations are marked in b by +, with each corresponding spectra shown in c . SERS spectra of AMP, adenosine and adenine (three representative spectra for each) were also measured for comparison ( d , see Methods for details). The horizontal axis shows Raman scattering shift in cm −1 . Probabilities for the occurrence of luminescence and SERS from fabricated regions are shown in e and f , respectively, for varying laser power, exposure time, cell type and HAuCl 4 concentration (1 or 2 mM). Error bars are not shown; probabilities are number of occurences divided by number of trials n where for HeLa cells, n =30 and for MH-S macrophages, n =15. Scale bar, 10 μm. Full size image The spatial resolution and molecular sensitivity of SERS detection is high enough that adjacent spectra are often very dissimilar, which produces highly variant spectra over distances as small as 50 nm [3] . In the sample shown in Fig. 6b , it is clear that luminescent spots produced by 5 mW and 5 s are the most likely to produce SERS signals. We estimated SERS generation in a variety of chemical and laser conditions for both endothelial HeLa cells and macrophage MH-S cells (6e), and found no significant dependence on cell type for these two cell lines. In summary, the creation of gold nanoparticles in cells leads to luminescent or SERS signals, with SERS being observed at a lower probability, presumably owing to the need for some amount of aggregation to occur. The clusters of small particles may be ideal for SERS since surface geometry can strongly influence the amount and localization of enhancement [27] . Mechanism and biological implications Biosynthesis of nanoparticles is known to occur in a number of different organisms [28] , and existing reports of longer-term (non light-based) reduction of gold ion solution inside cells [12] , [13] have been proposed to depend on cellular enzymes or processes. These processes occurring in cells should raise the overall background level of particles, but occur over longer time scales than the photoreduction results presented here, allowing us to confine the reduction to a laser focus region ( Figs 2a and 3a ). In bacteria, specific molecules involved with gold reduction have recently been identified [29] , while in non-biological environments, laser photoreduction to create metallic microstructures has been demonstrated and the corresponding reduction pathways are more amenable to experimental analysis [30] , [31] . While the photoreduction pathway in the cellular environment is not obvious, the results here show clearly that even with light, the presence of cellular components is required. Moreover, all measurements taken indicate the necessity of light, at least within time periods examined. It is therefore possible that previous reports of gold nanoparticle formation in cultured cells was in part due to the effects of ambient light over hours or days. The SERS detection aspect may also exhibit some nonlinear dependence on laser parameters ( Fig. 6f ), since SERS appeared only in the 2-mM results, and this would be consistent with the view that the SERS results from the degree of aggregation of small nanoparticles. While in the present implementation, long-term viability of cells is limited by high concentrations of HAuCl 4 , rapid damage of cells due to the acidity of the gold ion solution can be avoided by the phosphate buffers in the solution (see methods), which produce a final pH of 6–7. It is likely that harm to cells can further be mitigated by the use of gold caging or conjugation agents. In this context, it is important to remember that even in fixed cells, the temporal fluctuations of the SERS signal are significant [16] . The information gained from both point-based and line-based irradiation shows that particles can be fabricated anywhere in the cell with sufficient laser exposure, including the nucleus, while line irradiation highlights the existence of some spatial dependence in the fabrication mechanism. Taken together, these results show that gold ions penetrate the entire cell, but that the reduction process does retain some dependence on the local environment. The process is therefore mediated by local optical properties (that is, absorption) and by local structural or chemical properties. Since reduction requires an electron donor, the availability of such molecules, particularly those involved in cellular respiration such as NADH might provide a higher probability of photoreduction. Local pH conditions would be expected to affect the probability. The spatial dependence in Fig. 5 shows luminescence that appears stronger in cytosolic regions, where electron donors are more common. The spectral peaks in Fig. 6c are also somewhat similar to the spectra of adenosine and guanosine [24] , [32] , albeit with a peak shift towards the red of 20 cm −1 . With a large number of possible interactions with the myriad of intracellular molecules, the photoreduction pathways can be simplified by noting several key points. (1) Light is clearly the driving force, with spatial control of the reaction, (2) if the entire cell is irradiated, the luminescence signal is not homogenously distributed, as shown in Fig. 5 . This indicates that a dependence on both the irradiation field and the intracellular conditions is present, and (3) nanoparticle formation was not observed outside of the cells, showing that direct reduction of gold by 532-nm photons is not a significant pathway. Although photoreduction in a cell may in fact be simple, the exact pathway may be complicated to unravel. However, recently, a two-step photoreduction process was recently developed for photographic printing in gold [33] . Gold ion photoreduction played an important role as one of the most promising early techniques in photography, and in a collagen matrix, pure gold ion solution could be photoreduced to form images, given sufficient irradiation. However, the technique was too insensitive and was instead used as a later ‘toning’ step after irradiation of other photoreducable agents. Later, the use of simultaneous additional agents, notably iron (III)-based salts of citric, tartaric or oxalic acid [33] allowed the light-induced photoreduction of the additional ion to give high sensitivity, and in turn trigger the reduction of the gold ions in the same solution. The resulting multiple path reduction process depends on the concentration and type of additional ions present. In our experiments, any of the vast array of molecules in the cell could be photoreduced and then enable the reduction of the gold ions in the same manner, forming a type of intracellular chrysotype. Being able to modulate the amount or type of molecules, which are photoreduced in the cell that then lead to nanoparticles, would be an exciting future outcome of this work. The results of these experiments show that it is possible to fabricate gold nanoparticles with high reproducibility inside biological cells using gold ion solution and spatially selective light-driven growth. This allows the placement of particles anywhere in the cell by targeting an area of interest with a focused laser beam. Metallic particle-based laser fabrication of larger structures has previously been shown where particles are fused together, similar to sintering in metallurgy [31] , allowing the creation of arbitrary shapes. While the most useful metallic structure in a cell would appear to be nanoparticles, other shapes may be created and utilized in the future. Following this, we enscribed laser-targeted characters in the cell, showing a type of nano-tattoo that may find use in non-scientific applications, in the same way that a base of cultured cells in gold ion solution could find use as photographic-recording substrates. The most immediate applications, however, are the plasmonic applications of particles in cells. Nanometer-sized particles either singly, or in aggregation, enhance the electric field in the cell, amplifying the Raman signals from cellular molecules and allowing a unique method of probing the cell interior. The resulting SERS data show a variety of detected spectra, and many spectra contain peaks that are unique to that location. This emphasizes the importance of spatial resolution and targeted nanoparticle fabrication. In typical SERS measurements of a purified analyte, aggregation of nanoparticles is often intentionally induced since it changes the amount of detectable signal [24] . In the photoreduction process, the detection of SERS from fabricated regions likely occurs due to the growth of small particles, trapping biological molecules between particles, at hotspots in the enhanced field, creating ideal conditions for measurement. The variety of spectra generated demonstrates that there is indeed an abundance of molecular information available. It remains non-trivial, however, to classify and assign peaks to generated spectra. Even the first step of determining the location and quality of spectra requires an algorithmic approach, as we used here. Our approach did not use spectral signatures to isolate the presence of SERS spectra in the data, but rather ranked all spectra in terms of spectral energy and number or quality of peaks [19] . Expanding the spectral detection processing to include signatures of target molecules would be expected to assist the analysis of resulting data in future experiments. In addition, the creation of such small particle sizes is reported to limit the particle density of states and allow their use to catalyse organic reactions [34] , [35] , [36] . The direct fabrication process demonstrated here allows the particles to interact with the cell without capping agents or surface coatings, which block access to the gold surface. Results showing the luminescence contrast also hint that this technique can be used as a metal-based contrast agent. While the results shown here demonstrate the ability to measure intracellular targets using laser fabrication in the cell, further work is required to fully understand the nature of the molecular detection reported. Key issues are precisely which molecules are actually measured by the particles, and how the actual molecular distributions in the cell correspond to the measurements from the created probes. The ability of any surface-enhanced Raman technique to measure intracellular targets inherently lies in electromagnetic and chemical effects that combine to report Raman active molecules that are in nanoscale proximity to the surface. Direct estimation of the molecular distributions in the cell based on molecular signals reported by the particles is thereby complicated. Even assuming all cellular molecules are reported in 1:1 correspondence with their abundance at the laser focal point, and ignoring surface effects, Raman activity differences between molecules, and many other known issues, the nanoscale location of the particles will still affect the molecular signatures. It is interesting that the results reported here show different spectra to naked nanoparticles in a cell [16] , which are subject to endocytotic or other uptake pathways. This might simply be explained by the ability of the laser fabrication process to create particles at any location, but the results here also appear different to SERS measurements reported from the growth of nanoparticles in the cell over the course of several days incubation in cells without using light [13] . Whether these differences represent dependences on the particle locations, cell response or perhaps signify a fundamental difference in plasmonic properties of the particles in the different techniques is not known, and can only be elucidated by further studies. The photoreduction reaction occurs faster than many cell responses, so the induction of apoptotic or other pathways that drastically change molecular distributions in the cell can likely be neglected. It might also be possible to perform the photoreduction and SERS measurement simultaneously by using a Raman laser wavelength outside the luminescence region, to help clarify the temporal dynamics, if any, of the molecular signals. More refined control of the light-controlled reactions could be performed if caging and/or genetically encoding the requisite compounds for photofabrication is achieved. The TEM images show it is possible to produce a nearly diffraction-limited spot of nanoparticles, and the fabrication parameters ( Fig. 2 ) indicate a saturation effect. Saturation is a key to many super-resolution microscopy techniques, hinting that super-resolved fabrication may also be possible in the future. The most useful application is still, however, expected to be the generation of nanoparticles or metallic objects at target locations in a cell, not least because they allow the observation of molecular information from arbitrarily targeted regions selected by laser beam. Cell culture and treatment Cultured HeLa cells (93021013, PHE) were grown in Dulbecco’s modified Eagle’s medium (DMEM, Nacalai Tesque) supplemented with 10% foetal bovine serum, 2 mM glutamine, 100 units ml −1 penicillin and 100 μg ml −1 streptomycin, in a humidified atmosphere (5% CO 2 , 95% air) at 37 °C. For macrophage experiments, MH-S cells (CRL-2019, ATCC) were cultured in RPMI-1640 medium (Nacalai Tesque). Glass-bottomed culture dishes (Falcon) were used, except where TEM was performed, where plastic-bottomed dishes (Falcon) were used instead. In preparation for infusion of the gold ion solution, the culture medium was removed and cells were rinsed twice with phosphate-buffered saline. A bath solution of HAuCL 4 (Sigma) in phosphate-buffered saline at concentration ranges of between 0.5 and 2 mM was then added to the dishes and left to incubate at 23–25 °C for a period of time between 15 and 30 min. Following incubation cells were irradiated by 532-nm laser light. Unless otherwise noted, the gold ion solution was removed immediately following 532-nm irradiation. Photoreduction and spectroscopy Photoreduction was performed on a microscope observation stage in a clean room at 23 °C, using the 532-nm excitation laser of a Raman micro-spectroscopy system (Raman-11, Nanophoton). The excitation source was a semiconductor laser operating at 532 nm, with a power of up to 300 mW. The laser beam was focused into a point or line illumination pattern (selected by insertion of a cylindrical lens into the beam path) and irradiated the sample via a water-immersion objective lens (× 100/1.0 WI, Olympus). Scattered light was collected with the same objective and guided into a Czerny−Turner-type spectrometer with a focal length of 50 cm, and the final spectroscopic data were collected by an electrically cooled charge-coupled device camera (Pixis 400, Princeton Instruments). The overall spectral resolution was ~1.6 cm −1 , and optical resolution was ~400 nm. For measurement of luminescence from irradiated regions, the same 532-nm laser was used at lower power levels, which imaged the fabricated regions by the luminescence signal from gold. In addition, a 785-nm laser was used to measure Raman scattering from fabricated regions without exciting luminescence for measurement of SERS. Emitted light (either excited Raman scattering, autofluorescence or luminescence) was then collected by the same objective lens and guided to the spectrograph, and images were constructed using the wavenumber range 1,800–2,470 cm −1 . Image processing was done with ImageJ, and contrast quantification was done by a custom plugin, which integrates the change in intensity occurring in the laser focus region in the cell following irradiation. The surface-enhanced Raman spectral measurements were performed in a clean room at 23 °C, with the 785-nm laser focused across in a line across the whole field of view and each line of spectra were acquired with an exposure time of 1 s. The large amount of data requires some automation in the inspection, and therefore relevant spectra were extracted from the measured hyperspectral data stacks using ImageJ, following an analysis protocol we developed [19] . Briefly, spectra were mined by baseline correction then ranking all spectra according to the signal energy. Signals containing high ranking energy were then further graded based on number and quality of spectral peaks. Significant processing of the data occurs to detect and rank spectra, but after identifying the location of relevant spectra within the hyperstack, the final data output is not processed apart from baseline correction. Electron microscopy For TEM, 2.5% glutaraldehyde in 0.1 M Millonig’s phosphate buffer (NaH 2 PO 4 , NaOH, pH 7.3) was used. Cells were cultured on plastic culture dishes (Falcon) to enable later microtime operation. Cells were washed with 0.1 M Millonig’s buffer twice and then treated with 1% OsO4 in 0.1 M Millonig’s buffer for 1 h (4 °C). After 1 h, cells were washed in the same buffer and then treated with 0.15% tannic acid in buffer for 1 min. Cells were then washed once in the buffer, then twice in distilled water, stained with 1% uranyl acetate (4 °C) for 1 h and then washed in distilled water. This was followed by dehydration in a graded series of ethanol and embedded in Epoxy resin. Ultrathin sections were cut at a thickness of 70±5 nm and successive sections were laid on slotted copper grids with a support membrane coated by carbon. After staining with uranyl acetate and lead citrate, sections were viewed with TEM (H-7100, Hitachi, and Tecnai G2 F20 FE-TEM, FEI). Fabricated particle sizes were measured by HR-TEM, and particle composition was evaluated using energy-dispersive X-ray analysis. Nanoparticle-enhanced reference spectra acquisition Adenine-based compounds (adenine, adenosine and adenosine mono-phosphate) reference spectra were measured by dispersing 100 μl of a colloidal solution of 50 nm commercially sourced gold nanoparticles (EMGC50, BB International) onto a hydrophilic coated coverglass (MAS, Matsunami), allowed to stand for 2 min and then rinsed in distilled deionized water. Following drying, 20 μl of the 10-mM adenine-based solution was dispersed on the nanoparticle substrate. Following drying, reference spectra were measured by Raman imaging at 785 nm, with spectra of significance automatically evaluated using the same algorithm as for the photofabricated particle SERS data [17] . Simultaneous Raman/luminescence and phase imaging Simultaneous Raman/luminescence and quantitative phase imaging of the fabricated logo in the cells ( Fig. 4 ) was done with a custom system using a dichroic mirror-based separation of the Raman/luminescence region, with the quantitative absorption and phase measured by coherent excitation in a DHM imaging modality at 780 nm. Note that these imaging modes used 532 nm to excite Raman/luminescence and 780 nm to measure the phase. Further details are provided in a previous report [17] . To create a customized fabrication pattern in the cell, the laser focus was controlled by a set of x – y galvanometer mirrors (National Instruments), with the scan pattern imported as a binary array of points, translated into a raster pattern by software (Labview). DHM provides amplitude and phase; the absorption image is then calculated by squaring the amplitude. How to cite this article: Smith, N. I. et al . Laser-targeted photofabrication of gold nanoparticles inside cells. Nat. Commun. 5:5144 doi: 10.1038/ncomms6144 (2014).